Rational screening low-cost counter electrodes for dye-sensitized solar cells Dye-sensitized solar cells have attracted intense research attention owing to their ease of fabrication, cost-effectiveness and high efficiency in converting solar energy. Noble platinum is generally used as catalytic counter electrode for redox mediators in electrolyte solution. Unfortunately, platinum is expensive and non-sustainable for long-term applications. Therefore, researchers are facing with the challenge of developing low-cost and earth-abundant alternatives. So far, rational screening of non-platinum counter electrodes has been hamstrung by the lack of understanding about the electrocatalytic process of redox mediators on various counter electrodes. Here, using first-principle quantum chemical calculations, we studied the electrocatalytic process of redox mediators and predicted electrocatalytic activity of potential semiconductor counter electrodes. On the basis of theoretical predictions, we successfully used rust (α-Fe 2 O 3 ) as a new counter electrode catalyst, which demonstrates promising electrocatalytic activity towards triiodide reduction at a rate comparable to platinum. As one of the most abundant and yet least collected sources of renewable energy, solar energy has attracted considerable interest in scientific research and industrial applications. Dye-sensitized solar cells (DSCs) have stood out among various photovoltaic devices because of their low cost, relative high energy-conversion efficiency and simple production procedure [1] , [2] , [3] , [4] , [5] . In this rapidly developing field, finding active counter electrode (CE) material for triiodide reduction reaction (iodine reduction reaction) is of great importance for the promotion of DSCs. It has been confirmed that platinum (Pt) is a superior CE material with excellent catalytic activity, high electrical conductivity and stability. Unfortunately, the disadvantages such as the high cost and low abundance greatly restrict the large-scale application of Pt in DSCs [6] , [7] , [8] , [9] . Thus, several Pt-free alternative materials have been explored as CEs in DSCs, such as carbon materials [8] , [10] , conductive organic polymers [6] , [11] and inorganic semiconductor materials including metal sulfides [12] , [13] , metal nitrides [14] , [15] , metal carbides [16] , [17] , metal oxides [18] and copper zinc tin sulfide [19] and so on. Recently, Wu et al. [20] synthesized three classes (carbides, nitrides and oxides) of nanoscaled early-transition metal catalysts and applied them in DSC systems as CE catalysts to replace the expensive Pt. However, the rational screening for Pt-free alternative CE materials has not been explored, and the catalytic mechanism of electrocatalysis for triiodide reduction on the electrode surface has also not been fully understood so far. Herein, for the first time, we develope a general and efficient screening strategy for electrocatalytic activity of the potential non-Pt CE materials using first-principle calculations. Based on theoretical predictions, we explore a range of low-cost semiconducting materials, and successfully confirm that rust (α-Fe 2 O 3 ) nanocrystals mainly bounded by (012) and (104) surfaces demonstrate high electrocatalytic activity. The overall energy-conversion efficiency is comparable to that of Pt CE, and more importantly, the origin of the superiority of α-Fe 2 O 3 as the CE is investigated by kinetic analysis. Compared with Pt or some other CE materials, α-Fe 2 O 3 is composed of the most abundant elements in the Earth’s crust and has no toxicity. Thus, ferric oxide has superiority over other existing electrode materials in terms of the low cost, high abundance and superior efficiency. The findings in this work may pave the way for further development of more practical non-Pt CEs, which can help to accelerate the large-scale applications of DSCs in the future. Activity origin of Pt electrode and speculation To start a rational screening for the electrocatalytic activity of CE materials, it is essential to elucidate the origin of the excellent performance of Pt electrode for triiodide reduction, aiming at identifying the key parameter affecting the catalytic efficiency. Triiodide reduction reaction occurring on the CE can be written as: I 3 − (sol) +2e − →3I − (sol), and the general consensus of the reaction mechanism can be described as follows: I 3 − (sol)↔I 2 (sol)+I − (sol) (I) I 2 (sol)+2*→2I* (II) I*+e − →I − (sol) (III) where * represents the free site on the electrode surface and sol indicates the acetonitrile solution. The solution reaction, I 3 − (sol)↔I 2 (sol)+I − (sol), has been verified to be usually fast and considered to be in equilibrium [21] . The subsequent iodine reduction reaction (IRR: steps (II) and (III)) occurring at the liquid–solid interface, that is, the I 2 dissociation into two surface I atoms (I*) upon adsorption on the electrode surface and the removal of I* through one-electron transfer to produce solvated I − (sol), would determine the overall electrocatalytic activity. Herein, we first investigated these two elementary reactions at the interface of Pt(111) and CH 3 CN, CH 3 CN/Pt(111) (see Supplementary Note 1 for calculation model). To simulate the interface solution environment, several acetonitrile layers were introduced in the surface slab with a density of 0.79 gcm −3 , while the effect of electrode voltage on the material properties was taken into account by tuning the work function of Pt electrode [22] (see Supplementary Figs S1 and S2 ). Upon adsorption at the CH 3 CN/Pt(111) interface, iodine molecule can readily dissociate into two I* atoms, which sit preferably on the top of Pt atoms at a distance of d (Pt-I)=2.62 Å, giving rise to an adsorption energy of 0.52 eV at the CH 3 CN/Pt(111) interface (see Supplementary Note 2 ). For the one-electron reduction of I* into solvated I − (sol), the transition state with an elongated d (Pt-I)=4.20 Å was located, yielding a barrier as low as 0.39 eV under U eq =0.61 V versus SHE [23] , in favour of the kinetic feasibility. The standard Gibbs free-energy change of the half reaction (I 2 (sol)+2e − →2I − (sol)) was also calculated, being exothermic by 0.40 eV (see Supplementary Note 3 ). Therefore, IRR can be expected to proceed readily at CH 3 CN/Pt(111) interface. After obtaining the basic kinetic and thermodynamic data, we used the microkinetics to estimate the turnover frequency of the two-step reaction I 2 (sol)+2e − →2I − (sol) under the steady-state condition, the results of which show that IRR is determined by two important parameters, that is, I 2 dissociation barrier ( E a dis ) and I* desorption barrier ( E a des ). Moreover, it is found that E a dis and E a des are related to the adsorption energy of I ( E ad I ): E a dis is linear with E ad I with a negative slope ( E a dis =α 1 E ad I +β 1 , α 1 <0, a typical Bronsted–Evans–Polanyi relationship), whereas E a des increases linearly as E ad I goes up ( E a des =α 2 E ad I +β 2 , α 2 >0) on Pt(111) under different electrode voltages (see Supplementary Fig. S2 ). It is therefore clear that the binding strength of I on the Pt(111) has a crucial role in determining the catalytic activity in the reaction of I 2 (sol)+2e − →2I − (sol) (see kinetic analysis details in Supplementary Note 4 and Supplementary Fig. S3 ). These two linear relationships provide a kinetic base for placing the I adsorption energy as a fundamental property of rational screening, being in agreement with the rate-controlling rule obtained previously [24] , [25] . In other words, the adsorption energy of I atom on catalyst surfaces may be a good descriptor for the catalytic activity: Quantitatively, if the adsorption energy of I is too large, the desorption of I* into I − (sol) would be hard to proceed thermodynamically, limited by the large total Gibbs free-energy change of reaction (I*+e − →I − (sol)), and thus the overall activity is restricted; when I adsorption is weak, I 2 molecular dissociation is hindered. By virtue of density functional theory (DFT) calculations, we examined the adsorption of I atom on more than 20 candidate materials including metal oxides, carbide, nitride and sulphide, as summarized in Fig. 1a (see details in Supplementary Fig. S4 and Supplementary Table S1 ). It can be seen that the materials reported in the literature, such as WO 3 , CoS, NiS, FeS and TiN, possess adsorption energies around that of Pt [12] , [13] , [14] , [18] . On the other hand, of the unreported compounds, Cr 2 O 3 and Ta 2 O 5 may be expected to be less active owing to too strong M–I binding (M=Cr 3+ , Ta 5+ ), whereas the compounds such as TiO 2 , MnO 2 , SnO 2 , CeO 2 , ZrO 2 , La 2 O 3 , Al 2 O 3 and Ga 2 O 3 may be anticipated to possess limited activity because of their low binding ability towards I (being endothermic for I 2 dissociation). Ta 2 O 5 , TiO 2 and CeO 2 were selected to test experimentally and these predications are confirmed (see Supplementary Fig. S5 and Supplementary Table S2 ). Interestingly, Fe 2 O 3 (012) exhibits an almost identical adsorption energy of I with Pt (111) at the acetonitrile/electrode interface, indicating that it may be catalytically active. 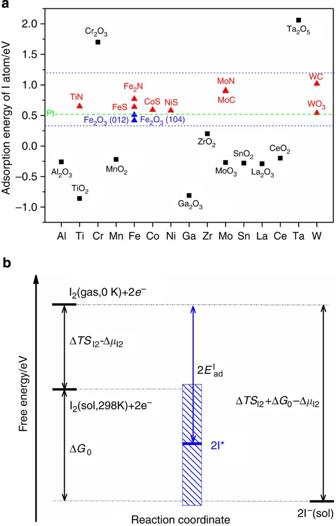Figure 1: Calculated adsorption energy of I atom on various compounds and framework to estimate the suitable range ofEadI. (a) Calculated adsorption energy of I atom in the gas phase or in the CH3CN solvent using DFT method. Red triangles indicate the reported active materials; blank squares represent the unreported materials, which were predicted to be less catalytically active. For materials on which the adsorption of iodine atom is endothermic, solvent effects were not considered any more. (b) Demonstration of range estimation model for the suitable electrodes in terms of the adsorption energy of I atom.TΔSI2is the entropy correction term of I2in gas phase, ΔμI2is chemical potential difference of I2molecule in between gas phase and CH3CN solvent at 298 K and ΔG0is the Gibbs free-energy change of half reaction I2(sol)+2e−→2I−(sol). Figure 1: Calculated adsorption energy of I atom on various compounds and framework to estimate the suitable range of E ad I . ( a ) Calculated adsorption energy of I atom in the gas phase or in the CH 3 CN solvent using DFT method. Red triangles indicate the reported active materials; blank squares represent the unreported materials, which were predicted to be less catalytically active. For materials on which the adsorption of iodine atom is endothermic, solvent effects were not considered any more. ( b ) Demonstration of range estimation model for the suitable electrodes in terms of the adsorption energy of I atom. T Δ S I2 is the entropy correction term of I 2 in gas phase, Δ μ I2 is chemical potential difference of I 2 molecule in between gas phase and CH 3 CN solvent at 298 K and Δ G 0 is the Gibbs free-energy change of half reaction I 2 (sol)+2e − →2I − (sol). Full size image Establishment and application of the screening framework Having obtained the results above, we are in the position to establish a quantitative or semi-quantitative framework to estimate the suitable range of E ad I for active CE materials. Kinetically, it is advantageous if the Gibbs free-energy of a sequential multistep reaction occurred on the solid catalyst surface decreases step by step, ensuring the overall reaction to proceed in the forward direction [26] . With respect to IRR, it demands the chemical potentials following , in which μ e is the chemical potential of electron and μ Ι* is defined as [26] where θ I* and θ * are the coverages of adsorbed I* and free site * on the catalyst surface, respectively; is the standard chemical potential of species I* and can be readily obtained from the adsorption energy of I from DFT with the necessary thermal correction. Cheng and Hu [26] proposed that the coverage-dependent term RT ln θ I* / θ * would lie in a small range on the best catalyst (about 0.06–0.12 eV at 298 K) and was defined as ε . Following the same approach, we can obtain the theoretical boundaries for the adsorption energy of I atom on good electrode surface (see Supplementary Note 5 ): in which is the entropy correction term of I 2 in gas phase at T=298 K (relative to gaseous I 2 at 0 K), is chemical potential difference of I 2 molecule in between gas phase and CH 3 CN solvent at 298 K and Δ G 0 ( ) is the Gibbs free-energy change of half reaction I 2 (sol)+2e − →2I − (sol). It should be noted that for clarity, we neglected the minor contribution of I 2 and I − concentration in the solution (~0.02 eV, estimated from experimental condition) to the free energy. Equation (2) sets two boundaries for I adsorption: The lower boundary requires that the binding strength between the electrode and I atom should be so strong that I 2 dissociative adsorption is exothermic in Gibbs free-energy, whereas the upper boundary ensures the subsequent desorption to proceed also exothermically, as shown in Fig. 1b . It is worth pointing out that the free-energy change Δ G 0 varies with the electrode voltage U that determines the electronic chemical potential μ e ( μ e = eU versus SHE). When (−0.06 V versus SHE), Δ G 0 reaches approximately maximum and thus provides the maximal upper boundary for E ad I according to equation (2). Therefore, to be inclusive, we estimated the variation range of E ad I under the condition U =−0.06 V versus SHE, which gives rise to the range from around 0.33 to 1.20 eV for good catalysts. Using this range to re-evaluate the above CE materials, we can see the usefulness of the adsorption range for catalyst screening, as shown in Fig. 1 . Some CE materials such as CoS, MoC, MoN, FeS, NiS, WC and WO 3 are known experimentally to be good catalysts ( Fig. 1a , red triangles) and possess a E ad I within the range, supporting the feasibility of this strategy. As an example, according to the theoretical calculations, the E ad I of CoS (0.59 eV) is closed to that of Pt (0.52 eV). Grätzel and co-workers deposited electrochemically CoS nanoparticles on PEN/ITO film to obtain a high-performance Pt-free CE [12] . The energy-conversion efficiency reached the same level of the Pt-CE DSCs, which matches well with the theoretical screening strategy shown in this work. For the materials, the activities of which remain to be tested, including TiO 2 , MnO 2 , SnO 2 , CeO 2 , ZrO 2 , La 2 O 3 , Al 2 O 3 , Ga 2 O 3 , Cr 2 O 3 and Ta 2 O 5 , E ad I are out of the optimal range ( Fig. 1a , black squares), indicating that their activity may be low. On two typical surfaces of α-Fe 2 O 3 , Fe 2 O 3 (012) and Fe 2 O 3 (104), E ad I are 0.51 and 0.42 eV, respectively, and they are within this estimated range for suitable CE materials. The activity comparison between α-Fe 2 O 3 and Pt electrode To further estimate the activity of Fe 2 O 3 , a detailed DFT calculation on the whole reaction pathway of IRR, involving the reaction barriers of I 2 dissociation and I* removal into I − (sol), was carried out at the interface of CH 3 CN/Fe 2 O 3 (012) and CH 3 CN/Fe 2 O 3 (104), respectively. The CH 3 CN/Fe 2 O 3 (012) interface model is illustrated in Fig. 2d . On both interfaces, it is found that I 2 molecules can dissociate directly and the formed I atoms sit on the top of five-coordinated surface Fe 3+ ions ( Fig. 2e ), whereas the desorption barrier of I* from the surface to CH 3 CN solvent was calculated to be as low as 0.18 and 0.08 eV on (012) and (104) surfaces, respectively. The transition state of I* desorption at CH 3 CN/Fe 2 O 3 (012) interface is shown in Fig. 2f , with a much elongated Fe–I bond length (4.12 Å) as compared with the initial Fe–I bond length (2.72 Å) in the adsorption configuration. The binding properties of Fe–I bond in the transition state were also investigated by virtue of charge density difference and Bader charge analysis (see Supplementary Fig. S6 ), indicating the ionic bond characteristic between Fe 3+ and ion-like I (with 0.69 e from Bader charge). Kinetically, as shown in Fig. 2g , the overall standard free-energy profiles on both Fe 2 O 3 (012) and (104) surfaces have no particularly high point. Therefore, it can be expected that Fe 2 O 3 (012) and Fe 2 O 3 (104) would exhibit kinetically good performance for the I 3 − reduction reaction. In addition, the energy level at the conduction band edge of Fe 2 O 3 (012) was calculated to be higher relative to the position of I 3 − /I − equilibrium potential, indicating the ability of Fe 2 O 3 in electron transfer to I 3 − (see Supplementary Fig. S7 ). To obtain a comparison further, we calculated the reaction profile of I 2 +2e − →2I − at CH 3 CN/Pt(111) interface, and the corresponding interface model, adsorption configuration of I* and transition state of I* desorption are illustrated in Fig. 2a–c . Comparing the whole reaction energy profile of Fe 2 O 3 with that on Pt electrode ( Fig. 2g ), the two Fe 2 O 3 surfaces have lower apparent barriers, suggesting that a higher catalytic activity for iodine reduction on α-Fe 2 O 3 CEs could be expected. 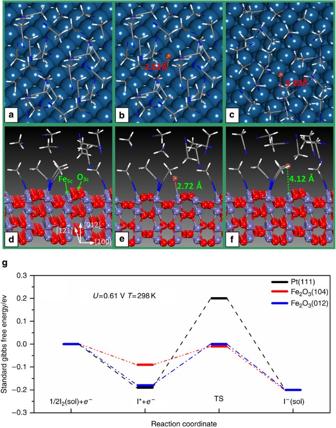Figure 2: The related structures involved in IRR and energy profiles. (a–c) Pt(111) surface structure in the presence of CH3CN solvent, I adsorption structure and the transition-state structure. (d–f) For the α-Fe2O3(012) surface, similar witha–c. (g) Energy profiles of the whole CE reaction on Pt(111), Fe2O3(104) and Fe2O3(012), respectively, which were calculated atU=0.61 V vs SHE. Figure 2: The related structures involved in IRR and energy profiles. ( a – c ) Pt(111) surface structure in the presence of CH 3 CN solvent, I adsorption structure and the transition-state structure. ( d – f ) For the α-Fe 2 O 3 (012) surface, similar with a – c . ( g ) Energy profiles of the whole CE reaction on Pt(111), Fe 2 O 3 (104) and Fe 2 O 3 (012), respectively, which were calculated at U =0.61 V vs SHE. Full size image Characterizations of α-Fe 2 O 3 and as-prepared CEs To verify these theoretical predictions, pure-phase Fe 2 O 3 was synthesized via a simple modified hydrothermal method using Iron (III) nitrate nonahydrate Fe(NO 3 ) 3 ·9 H 2 O and sodium-hydroxide aqueous solution as the precursor and the reaction controlling agent, respectively [27] . All diffraction peaks of the typical X-ray diffraction pattern (see Supplementary Fig. S8 ) match well with the crystal structure of the α-Fe 2 O 3 phase (space group: R-3c , JCPDS No. 84-0310). Representative electron microscopy images of α-Fe 2 O 3 nanoparticles and electrode films (cross-section) were shown in Fig. 3a . Square-like paticles were formed and these α-Fe 2 O 3 nanocrystals were mostly exposed by (012) and (104) facets. The enlarged transmission electron microscopy image shows the (012) and (104) planes with a lattice spacing of 2.68 Å and interfacial angle of 85° (ref. 28 ). To confirm the catalytic activity of the α-Fe 2 O 3 , subsequently, the as-prepared α-Fe 2 O 3 powder was used as CE materials to fabricate DSCs. 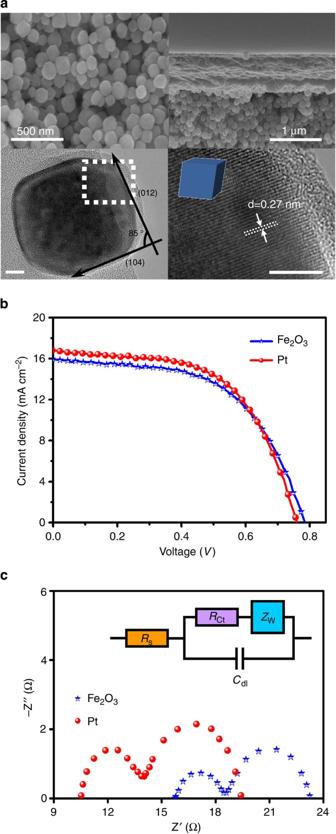Figure 3: Photocurrent–voltage curves and Nyquist plots from the impedance measurement. (a) The scanning electron microscopy images of α-Fe2O3nanoparticles and electrode films (cross-section) and the transmission electron microscopy images of α-Fe2O3nanoparticles. Scale bar, 5 nm. (b) Photocurrent–voltage (J–V) curves of DSCs with different CEs: α-Fe2O3(blue line) and Pt (red line), which were measured in the dark and under illumination of air mass 1.5 G full sunlight (100 mW cm−2). (c) Nyquist plots for the symmetric cells with two identical CEs of α-Fe2O3(blue) or Pt (red). The cells were measured with the frequency range from 100 MHz to 1 MHz, and the amplitude of the alternating current was set to 10 mV. The corresponding circuit is shown in the inset. Figure 3: Photocurrent–voltage curves and Nyquist plots from the impedance measurement. ( a ) The scanning electron microscopy images of α-Fe 2 O 3 nanoparticles and electrode films (cross-section) and the transmission electron microscopy images of α-Fe 2 O 3 nanoparticles. Scale bar, 5 nm. ( b ) Photocurrent–voltage ( J–V ) curves of DSCs with different CEs: α-Fe 2 O 3 (blue line) and Pt (red line), which were measured in the dark and under illumination of air mass 1.5 G full sunlight (100 mW cm −2 ). ( c ) Nyquist plots for the symmetric cells with two identical CEs of α-Fe 2 O 3 (blue) or Pt (red). The cells were measured with the frequency range from 100 MHz to 1 MHz, and the amplitude of the alternating current was set to 10 mV. The corresponding circuit is shown in the inset. Full size image Photovoltaic data Figure 3b demonstrates the photocurrent–voltage ( J–V ) curves for the DSCs and Nyquist plots of electrochemical impedance spectroscopy (EIS) for the dummy cells, respectively. The photovoltaic parameters are displayed in Table 1 . As shown in Fig. 3b , the short-circuit photocurrent density ( J sc ), open-circuit voltage ( V oc ) and fill factor of DSCs based on α-Fe 2 O 3 CE are 15.92 mA cm −2 , 784 mV and 0.56, respectively, yielding an overall energy-conversion efficiency (Eff.) of 6.96%, which is remarkably comparable to that of DSCs with Pt CE (7.32%). The results demonstrate that α-Fe 2 O 3 possessed an excellent catalytic activity to reduce oxidized triiodide to iodide. The observed low J sc with α-Fe 2 O 3 CE may be attributed to high resistance for electron transport owing to a thick film used (see Supplementary Fig. S9 ). Interestingly, a higher open-circuit voltage ( V oc ) with 25 mV of improvement was observed after replacing the Pt CE with α-Fe 2 O 3 CE. The photovoltaic results indicate that the α-Fe 2 O 3 shows a Pt-like catalytic behaviour. Table 1 Photovoltaic parameters of DSCs with different counter electrodes and the simulated data from EIS spectra. Full size table Electrochemical impedance spectroscopy To further investigate the electrochemical characteristics of α-Fe 2 O 3 electrodes, the EIS measurements were carried out with symmetric cells fabricated with two identical electrodes (CE//electrolyte//CE) at 20 °C. The Nyquist plots ( Fig. 3c ) illustrated impedance characteristics, in which two semicircles can be observed in the high-frequency (left) and low-frequency (right) regions. The high-frequency intercept on the real axis (Z′ axis) represents the series resistance ( R s ). The semicircle in the high-frequency regions arise from the charge-transfer resistance ( R ct ) [29] . In contrast to Pt, the larger R s and smaller R ct of the α-Fe 2 O 3 can be observed. The R s is mainly composed of the bulk resistance of α-Fe 2 O 3 , resistance of fluorine-doped SnO 2 (FTO) glass substrate, contact resistance and so on. The significant difference of R s between α-Fe 2 O 3 (15.8 Ω) and Pt (10.5 Ω) is obvious. The bulk resistance, conductivity of α-Fe 2 O 3 and adhesive between α-Fe 2 O 3 and FTO substrate should be responsible for its higher R s . With respect to photovoltaic performance and EIS fitting data, it can be deduced that R ct of CEs is a major factor in the performance of DSCs, suggesting catalytic activity for triiodide reduction [30] . In Table 1 , the R ct of α-Fe 2 O 3 is 2.3 Ω and this value is much smaller than the R ct of Pt (3.4 Ω), which may be one important cause that the energy-conversion efficiency of DSCs using α-Fe 2 O 3 CE is comparable to that of Pt CE. Thus, the high catalytic activity of α-Fe 2 O 3 is validated and a faster reduction rate of triiodide on the α-Fe 2 O 3 CE was obtained. The equivalent circuit used to fit the experimental EIS data is shown in the inset of Fig. 3c . In the modelling circuit used to mimic the EIS set up, the left semicircle consisting of R ct , C dl and Z w represents the CE [12] , [31] . Similar circuits have been used to model carbonaceous systems earlier [32] . C dl stands for the double-layer capacitance at the electrode/electrolyte interface because of the accumulation of ions at the electrode surface. The C dl indicates a surface property of the materials [16] . In the case of these two CE materials, the C dl of α-Fe 2 O 3 is 5.8 μF, indicating a similar surface area as compared with Pt (6.3 μF). Z w stands for Warburg impedance, which arises from mass transport limitations due to diffusion of the triiodide/iodide couple in the electrolytes [14] . Electrochemical behaviours It is well known that cyclic voltammetry (see Supplementary Fig. S10 ) and Tafel-polarization measurement are powerful electrochemical characterization methods. Fig. 4a demonstrates the Tafel-polarization curves of the symmetrical cells. They show the current density ( J ) as a function of voltage ( U ) at 20 °C for the oxidation/reduction of triiodide to iodide. The slope of a tangent to the α-Fe 2 O 3 curve is higher than that of Pt, indicating that α-Fe 2 O 3 shows a larger exchange current density ( J 0 ), which is also in good agreement with the EIS values in terms of the following equation (3) [12] , [33] . 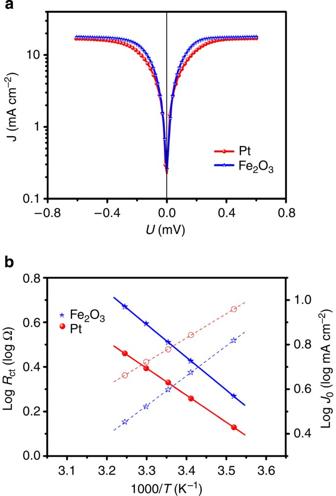Figure 4: Tafel-polarization curves and Arrhenius plots of LogRctand LogJoversus temperature. (a) Current–voltage characteristics of the symmetrical (CE//IL//CE) cells fabricated with two identical α-Fe2O3and Pt electrodes at 20 °C. (b) Charge-transfer resistance–temperature (left ordinate) and exchange current density–temperature data (right ordinate) in the Arrhenius coordinates with different CEs: α-Fe2O3(blue line) and Pt (red line). Figure 4: Tafel-polarization curves and Arrhenius plots of Log R ct and Log J o versus temperature. ( a ) Current–voltage characteristics of the symmetrical (CE//IL//CE) cells fabricated with two identical α-Fe 2 O 3 and Pt electrodes at 20 °C. ( b ) Charge-transfer resistance–temperature (left ordinate) and exchange current density–temperature data (right ordinate) in the Arrhenius coordinates with different CEs: α-Fe 2 O 3 (blue line) and Pt (red line). Full size image where R is the gas constant, T is the temperature, F is the Faraday’s constant and n is the number of electrons involved in the electrochemical reduction of triiodide at the electrode. These results confirm that the catalytic activity of α-Fe 2 O 3 is sufficient to catalyse the reduction of triiodide to iodide [21] . To further investigate the catalytic activity of the electrode materials, we scrutinized the variation tendency of the charge-transfer resistance and exchange current density in different temperature. Fig. 4b shows the logarithmic change-transfer resistance (Log R ct )—temperature (left ordinate) and logarithmic exchange current density (Log J 0 )—temperature data (right ordinate) in the Arrhenius coordinates. The exchange current density, J 0 , was calculated from impedance spectroscopy data to be 5.3 and 3.6 mA cm −2 at 20 °C for the α-Fe 2 O 3 CE and Pt CE, respectively. Compared with the Pt catalysts, the α-Fe 2 O 3 shows better catalytic activity for triiodide reduction, being consistent with the theoretical result given in Fig. 2g . The exchange current density ( J 0 ) shows temperature dependence ( Fig. 4b , right ordinate), following the Arrhenius equation (4) [12] : where I 0 is the exchange current density at T=infinite and E a is the activation energy. These results demonstrate that the electrochemical triiodide reduction reaction on the α-Fe 2 O 3 CEs is comparatively enhanced, which is in good accordance with the theoretical calculations. Therefore, α-Fe 2 O 3 can be expected to replace the expensive Pt in DSCs as a promising CE catalyst. In summary, using theoretical calculations, a general principle is developed in this report for screening Pt-free alternative CE materials for triiodide reduction reaction in DSCs. The screening principle not only offers a promising approach to advance the insight into the inherent catalysis on the CE materials but also helps to predict the new compounds that could serve as highly efficient CE materials. Importantly, this work also illustrates the power of combining first-principle calculations and experimental techniques to achieve the rational design of low-cost and high-efficiency CE materials for DSCs. DFT calculations All the spin-polarized calculations were performed with Perdew–Burke–Ernzerhof (PBE) functional within the generalized gradient approximation using the Vienna ab-initio simulation package code, unless otherwise specified [34] , [35] . The project-augmented wave method was used to represent the core-valence electron interaction. The valence electronic states were expanded in plane-wave basis sets with energy cutoff at 450 eV. The occupancy of the one-electron states was calculated using the Gaussian smearing for non-metal compounds and Methfessol–Paxton smearing for Pt(111). The ionic degrees of freedom were relaxed using the Broyden–Fletcher–Goldfarb–Shanno minimization scheme until the Hellman–Feynman forces on each ion were <0.05 eV Å −1 . The transition states were searched using a constrained optimization scheme [36] and were verified when (i) all forces on atoms vanish and (ii) the total energy is a maximum along the reaction coordination but a minimum with respect to the rest of the degrees of freedom. The force threshold for the transition-state search was 0.05 eV/Å. The dipole correction was performed throughout the calculations to take the polarization effect into account. With respect to some specific oxides, such as Fe 2 O 3 , MnO 2 and CeO 2 , it should be noted that one may consider other approaches for self-interaction correction, such as DFT+ U . However, DFT+ U presents its own limitations in terms of different U value that have to be chosen for the specific surface configurations or different oxide in principle, and thereby the results could be difficult to directly compare with. Herein, we checked the self-interaction corrections by utilizing hybrid functional HSE06 for Fe 2 O 3 , although it is very time-consuming. It showed that HSE06 gives an almost same barrier for the I* removal from the electrode surface (the rate-determining step) with that calculated using PBE functional, indicating that PBE may reasonably identify the reaction mechanisms. In addition, it should be noted that in the optimization of α-Fe 2 O 3 , we test the effect of spin state of d electrons in Fe 3+ , which showed that the high-spin antiferromagnetic arrangement is the most stable state and gives the lowest free energy [37] . To calculate the adsorption energy of surface species in the realistic solution, we take the effect of solvent implicitly into account by introducing several CH 3 CN solvent molecules into the surface model. The adsorption energy of I ( E ad I ) is defined as: where E (interface), E (I 2 ) and E (I/interface) are the energies of the liquid/electrode interface, I 2 in the gas phase and I adsorbed on the liquid/electrode interface, respectively. The larger E ad I is, the more strongly the species I binds on surface. Synthesis of α-Fe 2 O 3 Commercial iron (III) nitrate nonahydrate (4.04 g, ≥98.5%, Sinopharm) was dissolved in deionized water (33 ml) under stirring for 1 h. Then sodium-hydroxide aqueous solution (6 M) was added dropwise until the pH value of the mixed solution was 1.5 and then stirred for 30 min at 20 °C. Subsequently, the mixture was transferred into a Teflon-lined stainless autoclave and hydrothermally treated at 200 °C for 24 h. The product was cooled to room temperature by removing the heat source. Under ambient conditions, nanoparticles were separated by centrifugation at 9500, r.p.m. for 6 min and washed several times with deionized water and absolute ethanol. Electrode preparation The TiO 2 was prepared according to the literature [38] . A 12-μm thick layer of 20 nm-sized TiO 2 particles was loaded on the FTO conducting glass (Nippon Sheet Glass, Japan, 8 Ω per square) by screen printer technique. After sintering at 125 °C, the obtained layer was further coated with a 4-μm thick scattering layer of 200 nm-sized TiO 2 particles (DHS-NanoT200; Heptachroma) followed by sintering at 500 °C. After cooling to 80 °C, the two layers of TiO 2 films were immersed in a 5 × 10 −4 M solution of N719 dye (Solaronix SA, Switzerland) in acetonitrile/ tert -butyl alcohol (V/V=1/1) for 24 h. A total of 0.5 g α-Fe 2 O 3 powder was mixed with 2.03 g anhydrous terpineol, 2.6 g ethyl celluloses in ethanol (10 wt%) and 8 ml ethanol followed by stirring and sonication. The contents in dispersion were concentrated by evaporator, and then a layer of α-Fe 2 O 3 nanoparticles was loaded on the FTO conducting glass (NSG, 8 Ω per square) by screen printer procedure. The Pt electrode was prepared by drop-casting 0.5 mM H 2 PtCl 6 /ethanol solution on the clean FTO conductive glass. Subsequently, the FTO glasses coated with α-Fe 2 O 3 and Pt were then sintered in a muffle furnace at 450 °C for 30 min. Fabrication of DSCs DSCs were assembled together with the dye-sensitized TiO 2 electrode and the CE by a 25-μm thick hot-melt film (Surlyn 1702; DuPont) and sealed up by heating. The cell internal space was filled with electrolytes using a vacuum pump. The liquid electrolyte composed of 0.60 M 1-butyl-3-methylimidazolium iodide, 0.03 M I 2 , 0.50 M 4-tert-butyl pyridine and 0.10 M guanidinium thiocyanate with acetonitrile as the solvent. The sealed DSCs were used for the photocurrent–voltage test with an active area of 0.25 cm 2 . The symmetrical dummy cells used for EIS and Tafel-polarization measurement were assembled by two identical CEs, clipping the electrolyte similar to the one used for fabricating the DSCs. Material characterization The morphology and structure of the samples were characterized by high-resolution transmission electron microscopy (JEOL JEM-2010F, F20, 200 kV), field emission scanning electron microscopy (Hitachi S4800) and X-ray diffraction (Bruker D8 Advanced Diffractometer; Cu K α radiation; 40 kV). The current-voltage tests of DSCs were performed under one sun condition using a solar light simulator (Oriel 91160; air mass 1.5 G). The power of the simulated light was calibrated to 100 mW cm −2 using a Newport Oriel PV reference cell system (model 91150 V). The EIS experiments and Tafel-polarization curves were measured with dummy cells in the dark by using an electrochemical workstation (Parstat 2273; Princeton). The frequency range of EIS experiments was from 100 MHz to 1 MHz with an AC modulation signal of 10 mV and bias DC voltage of 0.60 V. The curves were fitted by the ZSimpWin software. Tafel-polarization measurements were carried out with a scan rate of 50 mV s −1 . Cyclic voltammetry was conducted in a three-electrode system in an acetonitrile solution of 0.1 M LiClO 4 , 10 mM LiI and 1 mM I 2 at a scan rate of 20 mV s −1 by using a BAS 100B/W electrochemical analyser. Pt served as a CE, and the Ag/Ag + couple was used as a reference electrode. How to cite this article: Hou, Y. et al. Rational screening low-cost counter electrodes for dye-sensitized solar cells. Nat. Commun. 4:1583 doi: 10.1038/ncomms2547 (2013).